Meta-analysis shows the impacts of ecological restoration on greenhouse gas emissions International initiatives set ambitious targets for ecological restoration, which is considered a promising greenhouse gas mitigation strategy. Here, we conduct a meta-analysis to quantify the impacts of ecological restoration on greenhouse gas emissions using a dataset compiled from 253 articles. Our findings reveal that forest and grassland restoration increase CH 4 uptake by 90.0% and 30.8%, respectively, mainly due to changes in soil properties. Conversely, wetland restoration increases CH 4 emissions by 544.4%, primarily attributable to elevated water table depth. Forest and grassland restoration have no significant effect on N 2 O emissions, while wetland restoration reduces N 2 O emissions by 68.6%. Wetland restoration enhances net CO 2 uptake, and the transition from net CO 2 sources to net sinks takes approximately 4 years following restoration. The net ecosystem CO 2 exchange of the restored forests decreases with restoration age, and the transition from net CO 2 sources to net sinks takes about 3-5 years for afforestation and reforestation sites, and 6-13 years for clear-cutting and post-fire sites. Overall, forest, grassland and wetland restoration decrease the global warming potentials by 327.7%, 157.7% and 62.0% compared with their paired control ecosystems, respectively. Our findings suggest that afforestation, reforestation, rewetting drained wetlands, and restoring degraded grasslands through grazing exclusion, reducing grazing intensity, or converting croplands to grasslands can effectively mitigate greenhouse gas emissions. Global temperature is approaching a threshold that will have irreversible consequences for the future of our Earth, mainly due to the increasing concentrations of atmospheric greenhouse gases (GHG) such as carbon dioxide (CO 2 ), methane (CH 4 ) and nitrous oxide (N 2 O) [1] . Over the last 220 years, global CO 2 concentrations increased from 283 to 419 parts per million (ppm), CH 4 increased from 750 to 1925 parts per billion (ppb), and N 2 O increased from 273 to 336 ppb [2] . Land-use change and ecosystem degradation have caused massive anthropogenic emissions of GHG and altered natural ecological ecosystems from net sinks to net sources [3] , [4] . Restoring the degraded ecosystems and converting lands back to healthy ecosystems has been proposed as a vital strategy for stabilizing the Earth’s climate [5] . To limit global warming below the 2 °C threshold, there is an urgent need to reduce atmospheric GHG concentrations by restoring degraded ecosystems such as forests, grasslands and wetlands [6] . Ecological restoration is the process of assisting the recovery of an ecosystem that has been degraded, damaged, or destroyed (Society for Ecological Restoration and Policy Working Group 2002). The United Nations (UN) has declared 2021-2030 as the ‘UN Decade on Ecosystem Restoration’ and calls on countries to meet commitments to restore one billion hectares of land. The Bonn Challenge and the New York Declaration on Forests have established ambitious targets to restore 350 million hectares of forests worldwide by 2030 [5] . Thus, systematically understanding the impacts of ecological restoration on GHG emissions is imperative for making better restoration policies and improving the Intergovernmental Panel on Climate Change (IPCC) guidance of GHG inventories. Forests occupy approximately 30% of the global land surface and play a crucial role in regulating the global carbon (C) cycle and reducing global warming [7] , [8] , [9] . A recent estimation reported that global forests maintained a net C sink of −7.6 Gt CO 2 e yr −1 , reflecting a balance between gross C removals (−15.6 Gt CO 2 e yr −1 ) and gross emissions (8.1 Gt CO 2 e yr −1 ) from deforestation and other disturbances, e.g., clear-cut, fire, windthrows, insects, etc [10] . Afforestation and reforestation could change biomass accumulation and alter soil biogeochemical, physical and hydrological properties, thereby affecting the GHG fluxes [9] , [11] , [12] , [13] . Previous work found that converting croplands to forests increased CH 4 uptake due to the decreased soil bulk density, and afforestation decreased N 2 O emissions due to the reduced nitrogen (N) substrate availability [11] . The conversion of grasslands to forests might decrease CH 4 emissions but increase N 2 O emissions [12] . Although many studies showed that afforestation could enhance the CO 2 sink function of ecosystems [10] , [14] , some studies observed that forest lands continued to act as a CO 2 source even after several years of afforestation [15] . These diverse results suggest that the magnitude and direction of GHG dynamics driven by forest restoration are highly uncertain and could be affected by multiple factors, including ecosystem types, restoration ways, and restoration age [12] , [16] , [17] . It is undoubtedly necessary to explore the general patterns and the major controlling factors of GHG emissions in the restored forests. Grassland ecosystems constitute approximately 40% of the terrestrial biosphere [18] , and natural grasslands are usually identified as efficient sinks of atmospheric CH 4 and CO 2 [19] , but sources of N 2 O [20] . Grassland degradation leads to changes in soil nutrient content, soil moisture, and plant composition, which influences the pattern of GHG emissions [21] , [22] . It has been found that grassland degradation might decrease CH 4 uptake by 40% [23] . However, whether grassland restoration can reduce GHG emissions is still inconclusive [19] , [24] . Previous work reported that grassland restoration increased C accumulation and enhanced CH 4 uptake [24] , but some studies found that grassland restoration might stimulate N 2 O and CO 2 emissions and shift grassland from a C sink to a C source [19] . Furthermore, the effects of grassland types, restoration measures, and restoration age on GHG emissions in the restored grasslands at a global scale are still unclear. Wetlands are considered to be one of the most efficient ecosystems for sequestrating CO 2 from the atmosphere [25] , mainly because inundation creates anaerobic conditions that prevent the decomposition of dead plant material and restore sequestered C in soil [26] , [27] . Despite covering only 5–8% of the Earth’s landscape, global wetlands store 20–30% of soil C on the Earth and thereby play an important role in the global C cycle [28] . In general, wetland drainage and degradation decrease CH 4 emissions but enhance CO 2 and N 2 O emissions to the atmosphere, converting the wetlands from C sinks into sources [29] , [30] . However, the impacts of restoration on wetland GHG and the driving factors remain controversial [31] , [32] , [33] . Previous work reported that wetland restoration could shift the ecosystems into net GHG sources [32] , [34] , [35] or net sinks [36] . The inconsistent results are probably attributed to the wetland restoration types, restoration age, climate, water table depth, and soil properties [32] , [37] . Since wetland restoration generally decreases CO 2 emissions but increases CH 4 emissions [32] , [34] , [36] , the overall effects of wetland restoration on the global warming potentials (GWP) considering three major GHGs (i.e., CO 2 , CH 4 , and N 2 O) are not well understood. Despite numerous studies investigating the effects of ecological restoration on the emission of individual or a few GHGs at the plot or regional level [38] , the general pattern of the impacts of ecological restoration on the three major GHGs at a global scale has not yet been analyzed. Furthermore, there is currently a lack of comprehensive global assessments for the three major ecosystems (i.e., forests, grasslands, and wetlands) which are crucial for the global GHG budget and the ‘UN Decade on Ecosystem Restoration’ [6] , [7] , [8] , [9] . In addition, detailed data on the responses of GHG to ecological restoration are lacking in the IPCC reports, the IPCC Guidelines for National Greenhouse Gas Inventories, and the Good Practice Guidance for Land Use, Land-Use Change and Forestry. To fill these knowledge gaps, we compiled a global dataset from 253 peer-reviewed articles and conducted a meta-analysis to assess the effects of ecological restoration on GHG emissions (Fig. 1 ). Our specific objectives were to (1) quantify the impacts of ecological restoration on CH 4 and N 2 O emissions and net ecosystem CO 2 exchange (NEE) in forest, grassland and wetland ecosystems, (2) explore the patterns of GHG emissions with restoration age, and (3) determine the key factors influencing the response of GHG emissions to ecological restoration. Fig. 1: Global distribution of the study sites for this meta-analysis. The free continental data of the world map was sourced from Natural Earth, supported by the North American Cartographic Information Society ( https://www.naturalearthdata.com/ ). ArcGIS Desktop 10.8 (Esri, West Redlands, CA, USA) was employed for mapping the distribution of the study sites. Source data are provided as a Source Data file. Full size image In this work, we show that forest and grassland restoration increases CH 4 uptake, mainly due to the changes in soil properties. Conversely, wetland restoration increases CH 4 emissions, primarily attributed to elevated water table depth. Forest and grassland restoration has no significant effect on N 2 O emissions, while wetland restoration reduces N 2 O emissions. Overall, forest, grassland and wetland restoration enhances C sink, reduces the global warming potentials, and can serve as strategies for mitigating GHG. Effects of ecological restoration on CH 4 emissions Overall, forest and grassland restoration significantly decreased CH 4 emissions, and the weighted response ratios ( RRd ) of CH 4 emissions were ‒2.3 (95% CI: ‒2.9 to ‒1.6) and ‒1.6 (95% CI: ‒2.4 to ‒0.8) under forest and grassland restoration, respectively (Fig. 2a ). Compared with the paired control ecosystems, forest and grassland restoration averagely increased CH 4 uptake from 1.0 to 1.9 kg C ha ‒1 year ‒1 (by 90.0%) and 2.6 to 3.4 kg C ha ‒1 year ‒1 (by 30.8%), respectively (Fig. 3b, c ). Among the types of grassland restoration, temperate steppe & meadow and desert steppe increased CH 4 uptake from 2.6 to 3.8 kg C ha ‒1 year ‒1 (by 46.2%) and 7.7 to 11.4 kg C ha ‒1 year ‒1 (by 48.4%), respectively (Fig. 3c ). Wetland restoration significantly increased CH 4 emissions by 544.4% ( RRd : 2.9; 95% CI: 2.4‒3.4; P < 0.05) (Fig. 2a ). The average CH 4 emissions increased from 23.4 kg C ha ‒1 year ‒1 to 150.8 kg C ha ‒1 year ‒1 after wetland restoration (Fig. 3a ). Among the types of wetland restoration, the conversion of grasslands to wetlands showed the largest increase in CH 4 emissions, with an average increase from 61.2 kg C ha ‒1 year ‒1 (in paired control) to 284.8 kg C ha ‒1 (in restored wetlands) (Fig. 3a ). In contrast, there was no significant change in CH 4 emissions when aquaculture ponds were converted to wetlands ( RRd : ‒1.7; 95% CI: ‒3.8 to 0.5) and mangroves were restored ( RRd : 1.1; 95% CI: ‒0.4 to 2.5) (Fig. 2a ). Fig. 2: Effects of ecological restoration on CH 4 (a), N 2 O (b), and NEE (c) fluxes across the different wetland, forest and grassland restoration categories. The overall effect size was calculated with a categorical random effects model. Values are means ±95% CIs of the weighted response ratios ( RRd ) between the paired control ecosystems and restored ecosystems. If the 95% CI value does not overlap with zero at the α = 0.05 level, the response is considered significant. The asterisks indicate significant positive or negative effects. Numbers next to the y-axis indicate sample sizes ( n ). Due to the small sample size for the paired restored-control measurements for the NEE in forests, the effects of forest restoration on the NEE were not tested by RRd . DG to W, drained grassland to wetland; DF to W, drained forest to wetland; DC to wetland, drained cropland to wetland, AQ to Wetland, aquaculture to wetland; NEE net ecosystem CO 2 exchange, TGM temperate steppe & meadow, AGM alpine steppe & meadow, DS desert steppe, AG artificial grassland. Source data are provided as a Source Data file. Full size image Fig. 3: Box plots of CH 4 and N 2 O fluxes in the restored wetlands and their paired control ecosystems (a and d), the restored forests and their paired control ecosystems (b and e), the restored grasslands and their paired control ecosystems (c and f). Every two adjacent boxes represent the paired control-restored measurements. The paired control ecosystems are prefixed with ‘P’. TGM, temperate steppe & meadow; AGM, alpine steppe & meadow. Box boundaries represent the 75th and 25th percentiles, whisker caps represent the 95th and 5th percentiles, and circle points represent outliers. Diamond points and solid lines inside the boxes represent means and medians, respectively. Asterisks (*) denote significance at p < 0.05, as determined by using a two-sided, independent samples t test. No adjustments were made for multiple comparisons. Numbers next to the x-axis indicate sample sizes (n). Exact p -values and Source data are provided as a Source Data file. Full size image Effects of ecological restoration on N 2 O emissions Overall, forest ( RRd : ‒0.4; 95% CI: ‒1.3 to 0.4) restoration did not affect N 2 O emissions, while grassland and wetland restoration reduced N 2 O emissions by 21.7% ( RRd : ‒0.7; 95% CI: ‒1.4 to ‒0.1) and 68.6% ( RRd : ‒2.9; 95% CI: ‒3.9 to ‒1.9; P < 0.05) (Fig. 2b ), respectively. When considering the types of forest restoration, the conversion of croplands to forests averagely decreased N 2 O emissions from 3.7 kg N ha ‒1 year ‒1 (in paired control) to 1.4 kg N ha ‒1 year ‒1 (in restored forests) ( RRd : ‒3.3; 95% CI: ‒4.7 to ‒1.9; P < 0.05) (Fig. 3e ). Among the types of wetland restoration (Fig. 2b ), the conversion of grasslands to wetlands averagely reduced N 2 O emissions from 5.2 kg N ha ‒1 year ‒1 (in paired control) to 2.6 kg N ha ‒1 year ‒1 (in restored wetlands), and the conversion of croplands to wetlands averagely decreased N 2 O emissions from 17.0 kg N ha ‒1 year ‒1 to 2.3 kg N ha ‒1 year ‒1 . Compared with the paired control ecosystems, peatland restoration averagely reduced N 2 O emissions from 2.2 kg N ha ‒1 year ‒1 to 0.5 kg N ha ‒1 year ‒1 . However, floodplains restoration did not significantly affect N 2 O emissions (Fig. 2b ). Among the measures of grassland restoration, the conversion of croplands to grasslands averagely decreased N 2 O emissions from 2.3 kg N ha ‒1 year ‒1 to 0.7 kg N ha ‒1 year ‒1 (Supplementary Fig. S1b ). Similarly, prairie restoration reduced N 2 O emissions from 4.8 kg N ha ‒1 year ‒1 to 0.1 kg N ha ‒1 year ‒1 ( RRd : ‒10.9; 95% CI: ‒14.7 to ‒7.1; P < 0.05 (Fig. 3f ). Effects of ecological restoration on CO 2 fluxes and GWP Overall, wetland restoration significantly reduced NEE by 138.8% ( RRd : ‒3.2; 95% CI: ‒3.8 to ‒2.5; P < 0.05) (Figs. 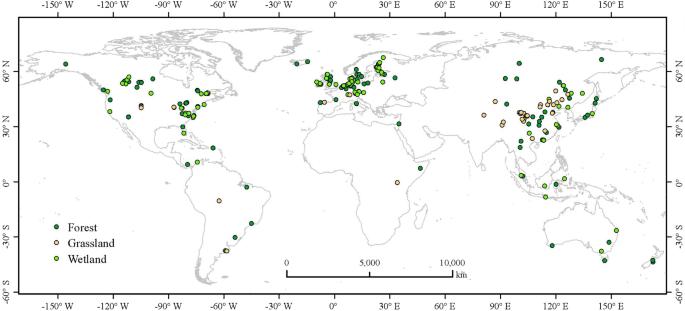Fig. 1: Global distribution of the study sites for this meta-analysis. The free continental data of the world map was sourced from Natural Earth, supported by the North American Cartographic Information Society (https://www.naturalearthdata.com/). ArcGIS Desktop 10.8 (Esri, West Redlands, CA, USA) was employed for mapping the distribution of the study sites. Source data are provided as a Source Data file. 2 c and 4a , Table 1 ). Compared with the paired control ecosystems, the conversion of grasslands to wetlands averagely reduced NEE from 231.9 g C m ‒2 year ‒1 to ‒219.5 g C m ‒2 year ‒1 , and the conversion of aquaculture to wetlands averagely reduced NEE from ‒41.9 g C m ‒2 year ‒1 to ‒151.5 g C m ‒2 year ‒1 (Supplementary Table S1 ). Bogs restoration averagely reduced NEE from 159.2 to ‒35.8 g C m ‒2 year ‒1 (Fig. 4a ). The conversion of grasslands to wetlands decreased gross primary productivity (GPP) and ecosystem respiration (ER), while bogs restoration increased GPP and ER (Supplementary Fig. S2 ). The floodplains and mangrove restoration showed no significant effect on GPP and ER (Supplementary Fig. S2 ). Fig. 4: Box plots of annual CO 2 fluxes (NEE, GPP and ER) the restored wetlands and their paired control ecosystems (a–c), the restored forests and their paired control ecosystems (d–f), and the restored grasslands and their paired control ecosystems (g–i). Every two adjacent boxes represent the paired control-restored measurements. The paired control ecosystems are prefixed with ‘P’. Box boundaries represent the 75th and 25th percentiles, whisker caps represent the 95th and 5th percentiles, and circle points represent outliers. Diamond points and solid lines inside the boxes represent means and medians, respectively. Asterisks (*) denote significance at P < 0.05, as determined by using a two-sided, independent samples t test. No adjustments were made for multiple comparisons. Numbers next to the x-axis indicate sample sizes (n). NEE net ecosystem CO 2 exchange, GPP, gross primary productivity, ER ecosystem respiration, TGM temperate steppe & meadow, AGM alpine steppe & meadow. Due to the small sample size for the paired restored-control measurements for the NEE, GPP, and ER in forests, the effects of forest restoration on CO 2 fluxes were not tested by the t-test. 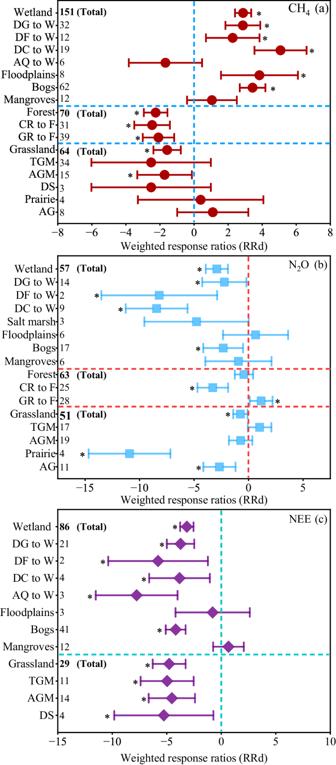Fig. 2: Effects of ecological restoration on CH4(a), N2O (b), and NEE (c) fluxes across the different wetland, forest and grassland restoration categories. The overall effect size was calculated with a categorical random effects model. Values are means ±95% CIs of the weighted response ratios (RRd) between the paired control ecosystems and restored ecosystems. If the 95% CI value does not overlap with zero at theα= 0.05 level, the response is considered significant. The asterisks indicate significant positive or negative effects. Numbers next to the y-axis indicate sample sizes (n). Due to the small sample size for the paired restored-control measurements for the NEE in forests, the effects of forest restoration on the NEE were not tested byRRd. DG to W, drained grassland to wetland; DF to W, drained forest to wetland; DC to wetland, drained cropland to wetland, AQ to Wetland, aquaculture to wetland; NEE net ecosystem CO2exchange, TGM temperate steppe & meadow, AGM alpine steppe & meadow, DS desert steppe, AG artificial grassland. Source data are provided as a Source Data file. Exact p -values and Source data are provided as a Source Data file. Full size image Table 1 Changes in comprehensive C budget and GWP when converting the paired control ecosystems to the restored ecosystems (Mean ± SE) Full size table Overall, grassland restoration decreased NEE by 146.9% ( RRd : ‒4.7; 95% CI: ‒5.8 to ‒3.5; P < 0.05) (Figs. 2 c, 4h and Supplementary Fig. S1c ). Compared with the paired control ecosystems, grassland restoration by grazing exclusion averagely decreased NEE from ‒245.3 g C m ‒2 year ‒1 to ‒703.0 g C m ‒2 year ‒1 , grassland restoration by reducing grazing density averagely reduced NEE from ‒587.9 g C m ‒2 year ‒1 to ‒1460.1 g C m ‒2 year ‒1 , and the conversion of cropland to grassland averagely reduced NEE from 10.3 g C m ‒2 year ‒1 to ‒75.8 g C m ‒2 year ‒1 (Supplementary Fig. S1c , Table S2 ). Grassland restoration increased GPP and ER (Supplementary Fig. S2 ). Due to the small sample size for the paired restored-control measurements for the NEE, GPP, and ER in forests, the effects of forest restoration on CO 2 fluxes were not tested by the RRd and t-test (Figs. 2 c, 4d–f ). Based on the restoration chronosequence sub-dataset, the NEE in restored forests decreased first and then tended to be stable and showed a negative exponential relationship with afforestation age, while the GPP and ER showed a positive exponential relationship with afforestation age (Fig. 5e ; P < 0.001). Similarly, the NEE was negatively and exponentially correlated with reforestation age and time since restoration after disturbance (Fig. 5f, g ; P < 0.001). Fig. 5: Relationships of the response ratios ( RRd ) of CH 4 and N 2 O fluxes, and the annual CO 2 fluxes with restoration age. a , b relationships between the response ratios of wetland CH 4 ( a ) and N 2 O ( b ) fluxes and restoration age. c Relationship between the response ratios of forest and grassland CH 4 fluxes and restoration age. d – f relationships between the CO 2 fluxes in wetland ( d ) and forest ( e and f ) and restoration age. g relationships between the fluxes of NEE and restoration age. h , i relationships between GPP/ER and afforestation time ( h ), and restoration age after forest disturbance ( i ). Linear and nonlinear regression were used and the error bands surrounding the regression lines represent the 95% confidence interval of the correlation. The n is the number of observations. Exact p -values and Source data are provided as a Source Data file. Full size image On average, the C budget (CO 2 and CH 4 ) was −295.5, −506.5 and −53.4 g C m −2 year −1 for forest, grassland and wetland restoration, respectively, indicating the capacity of enhanced C sink in the restored ecosystems (Table 1 ). On average, forest, grassland and wetland restoration decreased the GWP by 327.7%, 157.7% and 62.0% compared with their paired control ecosystems, respectively (Table 1 ). Changes of CH 4 and N 2 O emissions and NEE with restoration age Given the critical impact of restoration age on GHG emissions in restored ecosystems, the patterns of CH 4 and N 2 O emissions and NEE with restoration age were first explored. Overall, the restoration age had a significant effect on CH 4 emissions (Fig. 5c and Supplementary Fig. S3b ). The RRd of CH 4 emissions in the restored forests was negatively correlated with restoration age (i.e., years since restoration) (Fig. 5c ). The soil CH 4 uptake showed no response to the afforestation age within 10 years, while soil CH 4 uptake increased with afforestation age for longer time intervals (Supplementary Fig. S3b ). The RRd of CH 4 emissions in the restored wetlands was exponentially and positively correlated with restoration age and achieved a relatively stable value in about 10 years since restoration (Fig. 5a ). The RRd of N 2 O emissions in the wetland was negatively correlated with restoration age (Fig. 5b ). Restoration age was an important factor influencing CO 2 fluxes (Fig. 5 ). The GPP/ER showed low values (<1 or ≈1) in the early years following afforestation and restoration from fire and clear-cutting (Fig. 5g, h ). The GPP/RE became greater than 1 (i.e., NEE < 0) by 4 years, 6 years, 13 years, and 8 years after restoration for the afforestation sites, clear-cutting sites, post-fire sites, and all disturbances sites, respectively (Fig. 5 ). The GPP/ER ratio varied with afforestation age and time since restoration after disturbance, and had an asymptote of 1.19 and 1.09, respectively (Fig. 5g, h ; P < 0.001). The NEE in the wetlands was exponentially and negatively correlated with restoration age and the switchover time from net CO 2 sources to net CO 2 sinks was estimated to be approximately 4 years (Fig. 5d ). Factors influencing the response of CH 4 , N 2 O, and NEE to ecological restoration Forest restoration significantly increased concentrations of soil organic C (SOC), NH 4 + -N and dissolved organic C (DOC), but reduced soil temperature, soil water-filled pore space (WFPS), soil moisture, and pH ( P < 0.05; Fig. 6b ). Grassland restoration remarkably increased soil WFPS, soil moisture, vegetation coverage, and grassland aboveground and belowground biomass, but reduced soil bulk density (BD) and soil NO 3 ‒ -N concentrations ( P < 0.05; Fig. 6c ). Wetland restoration significantly increased water table depth, soil SOC and total N (TN), but decreased soil BD, soil redox potential (Eh), pH and NH 4 + -N concentrations ( P < 0.05; Fig. 6a ). Fig. 6: Effects of ecological restoration on soil properties in wetland (a), forest (b), and grassland (c) ecosystems. The overall effect size was calculated with a categorical random effects model. Values are meant ±95% CIs of the weighted response ratios ( RRd ) between the paired control ecosystems and restored ecosystems. If the 95% CI value does not overlap with zero, the response is considered significant. The asterisks indicate significant positive or negative effects. SOC soil organic carbon, TN total N, C: N carbon/nitrogen ratio, Eh soil redox potential, BD bulk density, SM soil moisture, WFPS water-filled pore space, ST soil temperature, WT water table depth, VC vegetation coverage, TB total biomass, AB aboveground biomass, BB belowground biomass; NH 4 + ammonium, NO 3 − nitrate. Source data are provided as a Source Data file. Full size image The RRd of CH 4 emissions in the restored forests was positively correlated with the RRd of soil WFPS ( P < 0.01; Fig. 7b ). The RRd of CH 4 emissions in the restored forests and grasslands was negatively correlated with the RRd of BD (Fig. 7a ). Afforestation decreased CH 4 emissions regardless of the tree types (i.e., coniferous and deciduous forest) ( P < 0.01; Supplementary Fig. S3c ). The RRd of N 2 O emissions in the forests and grasslands were positively correlated with the RRd of soil NH 4 + -N and NO 3 ‒ -N concentrations (Fig. 7d, e ), and the RRd of N 2 O emissions in the forests was negatively correlated with the RRd of soil pH ( P < 0.01; Fig. 7f ). Fig. 7: Relationships of the response ratios ( RRd ) of CH 4 (a–c), N 2 O (d–g), and NEE (h and i) with response ratios ( RRd ) of soil properties after wetlands, forest, and grassland ecosystems were restored. WT water table depth, BD bulk density, SM soil moisture, WFPS water-filled pore space, AB aboveground biomass, VC vegetation coverage. Linear and nonlinear regression were used and the error bands surrounding the regression lines represent the 95% confidence interval of the correlation. The n is the number of paired observations. Exact p -values and Source data are provided as a Source Data file. Full size image The RRd of CH 4 emissions in the restored wetlands was exponentially and positively correlated with water table depth ( P < 0.01; Fig. 5a and Fig. 7c ). The RRd of N 2 O emissions in the wetland was positively correlated with the RRd of soil NH 4 + -N concentrations (Fig. 7g ). The N 2 O emissions and NEE of the restored wetlands were negatively related to water table depth ( P < 0.001; Supplementary Fig. S4c ). Across all restoration groups, GPP and ER were positively correlated with the temperature and precipitation ( P < 0.01; Supplementary Fig. S5 ). The RRd of CH 4 emissions in all systems was negatively correlated with the aridity index ( P < 0.01; Supplementary Fig. S6c ). When the precipitation was larger than 900 mm, the RRd of N 2 O emissions in all ecosystems was positively correlated with precipitation ( P < 0.05; Supplementary Fig. S6e ). The RRd of NEE in all ecosystems was negatively correlated with the aridity index when the aridity index was greater than 0.9 ( P < 0.05; Supplementary Fig. S6i ). Forest and grassland restoration increased CH 4 uptake while wetland restoration enhanced CH 4 emissions We found that forest and grassland restoration significantly increased CH 4 uptake (Table 1 , Fig. 2 ), suggesting the great potential of forest and grassland ecosystem restoration in enhancing sink function for CH 4 . The conversion of croplands and grasslands to forests increased CH 4 uptake by 84.8% and 106.8% (Fig. 3 ), respectively, indicating high CH 4 removal efficiency. The RRd of CH 4 emissions linearly increased with the RRd of WFPS (Fig. 7b ), indicating that lower soil moisture and WFPS enhanced CH 4 uptake and inhibited CH 4 emissions from soil. Afforestation significantly decreased WFPS in the forest ecosystems (Fig. 6b ), mainly because trees had deeper roots and higher water demands than crops and grasses, and afforestation enhanced evapotranspiration and canopy interception of precipitation [39] , [40] . The decrease in soil WFPS caused by afforestation can enhance the diffusion of atmospheric O 2 and CH 4 into the soils, thereby increasing CH 4 oxidation and uptake in the afforested soils [39] . Soil compaction by machinery in the agricultural lands and trampling by livestock in the grasslands may increase soil bulk density and reduce soil porosity [41] , [42] , [43] . Our results showed that grassland restoration significantly reduced soil bulk density (Fig. 6c ), and the RRd of CH 4 emissions showed a negative relationship with the RRd of soil bulk density (Fig. 7a ), implying that the lower soil bulk density in the restored grasslands increased CH 4 diffusion from atmosphere into soils and thus increased CH 4 uptake [44] . Grassland restoration by reducing grazing intensity or grazing exclusion increased belowground biomass (Fig. 6c ), which may form “root holes” and improve soil aerobic conditions for diffusion of atmospheric CH 4 into the soil profiles and the growth of methanotrophs [45] , thereby enhancing CH 4 uptake in the restored grassland. In addition, the increase in SOC in the afforested lands (Fig. 6b ) could enhance soil macropores and the number of coarse pores [46] , and thus create favorable environments for methanotrophs growth and CH 4 oxidation [47] . Taken together, the increased CH 4 uptake in the restored forests and grasslands could be attributed to the changes in soil properties. Forest restoration significantly increased CH 4 uptake with the increase of afforestation age (Fig. 5c and Supplementary Fig. S3b ), which could be mainly attributed to the increased SOC and decreased soil moisture and WFPS following afforestation (Figs. 6 b and 7b ) [48] , [49] . Bárcena et al. reported that soil SOC concentrations increased with stand age and therefore increased the abundance and activity of methane-oxidizing bacteria growth by supplying abundant substrates [50] , consequently resulting in an enhanced CH 4 oxidation rate with afforestation age. Gatica et al. found that, with the increase of afforestation age, soil moisture was decreased by the combined effects of increasing rainfall interception [51] and tree transpiration in the older forest stands [39] , and thus enhanced CH 4 consumption with time. Therefore, these individual observations support our results and inferences [48] , [49] , [50] , [51] . We found that wetland restoration significantly increased annual CH 4 emissions by 5.4 times compared with the paired control ecosystems, indicating that wetland restoration enhanced the CH 4 source strength. Among the types of wetland restoration, the conversion of grasslands to wetlands showed the largest increase in CH 4 emissions, followed by the conversion of croplands to wetlands (Fig. 3a ). These results indicated that greater attention should be paid to the increased CH 4 emissions from the restored wetlands in global GHG accounting. Previous work showed that CH 4 emissions in the wetlands were mainly controlled by water table level [26] , [38] , nutrient status [44] , plant species [52] , and microbial activity [53] . Unlike the CH 4 emissions in forest and grassland ecosystems which were influenced by soil properties (Fig. 7a, b ), the RRd of wetland CH 4 emissions was positively correlated with water table depth, suggesting that the wetland restoration facilitated the production of CH 4 by creating an anaerobic environment through elevated water table levels (Figs. 6 a, 7c ). Long-time waterlogging during the restoration period reduced O 2 penetration into the sediments and thus induced a reduction in the redox potential of 1.23-fold compared with the paired control ecosystems (Fig. 6a ), which in turn stimulated methanogen growth and activity, thereby enhancing CH 4 emissions [54] . Bog restoration by rewetting may be beneficial to the proliferation of aerenchymatous vascular plants, and thus allow CH 4 to bypass the oxidized surface soil, consequently enhancing CH 4 emission into the atmosphere via the plant-mediated transport [32] . In addition, restoration of wetlands by rewetting created an anaerobic environment which may inhibit microbial activity and reduce SOC decomposition [55] , thus leading to a higher SOC concentration in the restored wetlands (Fig. 6a ). The higher SOC concentrations in the restored wetlands could provide more substrates for methanogen growth than in the paired control ecosystems [44] , [56] . Thus, elevating the water table level and increasing the substrate supply for methanogen is likely to result in higher CH 4 fluxes in the restored wetlands (Figs. 6 a, 7c , and Supplementary Fig. S4a ). The RRd of wetland CH 4 showed exponentially relationship with restoration age and achieved a relatively stable value in about 10 years since restoration (Fig. 5a ). Similarly, Mitsch et al. reported that wetland restoration initially stimulated CH 4 emissions but decreased over time and reached CH 4 emissions comparable to the natural wetland after 13-15 years [28] . The rapid response of CH 4 emissions to wetland restoration at the initial stage was mainly due to the restoration of the natural hydrology and the inundation of easily decomposable plant litters, which created an anaerobic environment and sufficient substrate for the growth of methanogens and CH 4 production [53] , [57] , [58] , [59] . Diverse responses of N 2 O emissions to ecological restoration Our findings revealed that the conversion of agricultural lands to forests significantly decreased N 2 O emissions and the conversion of grasslands and wetlands to forests stimulated N 2 O emissions, indicating the response patterns of N 2 O emissions to forest restoration depends on the prior land-use type. The RRd of N 2 O emissions in forests was positively related to the RRd of NH 4 + and NO 3 ‒ (Fig. 7 ), indicating that the cessation of fertilization in the afforested croplands may lead to a reduction in soil N 2 O emissions compared with the fertilized croplands [11] . The main reasons for the increased N 2 O emissions in the forests converted from grasslands could be attributed to that afforestation in grasslands increased the concentrations of soil SOC and NH 4 + and decreased soil pH (Fig. 7 , Supplementary Fig. S7 ). The increased SOC and NH 4 + could increase soil C and N availability and soil nitrification for N 2 O production [12] , [60] . Our results demonstrated that the RRd of N 2 O emissions showed a negative relationship with the RRd of soil pH (Figs. 6 b, 7f ). The reduction of soil pH may inhibit the activity of the N 2 O reductase enzyme and in turn increase N 2 O/N 2 ratios in the denitrification, consequently increasing N 2 O emissions from denitrification in the afforested soils [4] , [61] . Grassland restoration by conversion of cropland to grassland sharply decreased N 2 O emissions (Supplementary Fig. S1b ), mainly due to the decreased concentrations of soil NO 3 ‒ by stopping fertilization (Figs. 6 c, 7 ). In contrast, artificial assisted restoration in the degraded grasslands by applying organic or mineral fertilizer may increase N 2 O emissions by increasing the availability of N for N 2 O production [62] . Thus, our results indicated that different grassland restoration measures showed distinct impacts on N 2 O emissions (Supplementary Fig. S1b ). Wetland restoration significantly decreased N 2 O emissions (by 68.6%) and soil NH 4 + concentration, and the RRd of N 2 O emissions in wetlands was positively related to the RRd of NH 4 + (Figs. 2 b, 3 d, 6 a, 7g ), indicating that the reduction in soil NH 4 + concentration, driven by wetland restoration, contributes to the decreased N 2 O emissions in the restored wetlands (Fig. 6a ). Previous work showed that the conversion of agricultural lands and grasslands to wetlands significantly decreased N fertilizer and animal waste inputs, thus reducing the substrates of inorganic N for nitrifying and denitrifying microorganisms [63] . Raising the water table in rewetted peatlands can potentially increase the diffusional barrier for deep soil N 2 O emissions into the atmosphere and enhance the microbial complete reduction of N 2 O to N 2 by denitrifying bacteria [30] , [64] , [65] , thereby reducing N 2 O emissions in the restored peatlands [30] . In addition, Brummell et al. attributed the reduction of N 2 O emissions in the restored peatlands to the rapid reestablishment of vascular plants [66] , which effectively take up soil N by plant roots and thereby decrease N availability for nitrification and denitrification. Therefore, reducing soil N availability and raising water levels could create unfavorable environments for N 2 O emissions. Forest, grassland, and wetland restoration enhances C sink and reduces the GWP Our results demonstrated that the NEE decreased with afforestation and reforestation age, and the estimated time required for the transition from CO 2 sources to net sinks was approximately 3-5 years (Fig. 5 ), indicating that restored forests have the capacity to rapidly become CO 2 sinks. At the early stage of restoration, forests may act as weak CO 2 sources (Fig. 5 ), primarily due to the low foliar biomass and the rapid decomposition of residuals in the ground and soils [17] . As trees grow, the increases in GPP surpassed the rise in ER. The enhanced ability of C assimilation and the subsequent increase in annual woody biomass production are the key factors driving restored forests to function as CO 2 sinks [67] , [68] , [69] . The estimated switchover time of restored forests from CO 2 source to net sink after the disturbance was approximately 6 years for the clear-cutting sites and 13 years for the post-fire sites (Fig. 5 ), indicating a relatively slow recovery of the C sink function in the burned sites. Forest restoration progressively increased the GPP/ER ratio with restoration age, eventually reaching a stable value of 1.1-1.2 after approximately 20 years. Interestingly, this value aligns with the average GPP/ER ratio of 1.2 observed in mature forests worldwide [70] . Grassland restoration markedly reduced the NEE (Fig. 2c ), suggesting that grassland restoration effectively increased C sink capacity. The RRd of NEE in grassland was positively related to the RRd of soil moisture (Fig. 7h ), indicating that higher soil moisture increased grassland CO 2 sinks. Grassland restoration by grazing exclusion or reducing grazing density is conducive to the recovery of grassland and the increase of vegetation coverage (Fig. 6c ), thereby reducing evaporative water loss from the soil [71] . The increase in soil moisture in the restored grassland decreased NEE by increasing GPP relatively more than ER [72] . The results are consistent with the general observations that higher soil water content increased vegetation leaf area index and GPP, and thereby resulted in a great C sink capacity in the grassland ecosystems [73] . In addition, the significant relationship between grassland NEE and aboveground biomass suggested that grassland restoration by grazing exclusion favored the regrowth of grasses and increased above- and belowground biomass (Figs. 6c and 7h ), and thus increased gross ecosystem photosynthesis and eventually resulted in a significant decrease in NEE [74] . Grassland restoration by converting cropland to grassland remarkably decreased NEE (Supplementary Fig. S1c ), indicating an increased C sink. The large residual of dead roots in the soil with cropland harvest would decompose and release large CO 2 emissions, while the grassland had a large live root and thereby decreased ecosystem respiration and increased net CO 2 uptake in the grassland systems [75] . Therefore, the enhanced CO 2 uptake in the restored grassland was mainly due to the increase in soil moisture and vegetation biomass (Figs. 6 c, 7h ). Overall, wetland restoration significantly reduced the NEE and shifted the ecosystems into CO 2 sinks (Fig. 4a ), highlighting the effectiveness of wetland restoration in enhancing CO 2 sequestration. The significant negative correlation of NEE with water table depth in the restored wetlands indicated that the rise of the water table plays a crucial role in promoting the CO 2 sink (Supplementary Fig. S4c ). This pattern is expected since individual observations have confirmed that restoring the drained bog by raising the water table could create suitable conditions for vegetation growth, and the recolonization of bryophytes and vascular plants in restored wetlands contributed to the net CO 2 uptake [26] , [27] , [29] . Returning aquaculture to wetland significantly enhanced CO 2 sinks (Fig. 2c ), which may be mainly due to the increase of the aquatic vegetation biomass and the shift of dominant species from submerged vegetation to flotation vegetation [76] . In addition, we found that the NEE of wetlands showed a negative exponential relationship with restoration age, and the transition time from net CO 2 sources to net CO 2 sinks was estimated to be around 4 years (Fig. 5d ). Similarly, Waddington et al. reported that the restored peatlands could serve as net C sinks (20 g C m ‒2 ) after two years restoration, mainly due to the rapid increase in moss cover and biomass after rewetting [77] . Lee et al. reported that the eighth year of the restored peatlands exhibited a net C sink (163 g C m −2 yr −1 ) [78] , falling within the range of C sink values reported for pristine peatlands (50-267 g C m −2 yr −1 ) [26] , [79] , [80] , [81] . Over longer time frames, we can anticipate a gradual stabilization of the CO 2 sink as the biomass pool in the restored wetland approaches a steady C sequestration rate. Regarding the C balance (excluding DOC fluxes), wetland restoration increased CH 4 emissions and CO 2 uptake, resulting in net sinks with a mean of 53 g C m −2 yr −1 (Table 1 ). The balance between CO 2 sinks and the strong warming potentials of CH 4 and N 2 O emissions strongly determined the net climatic impact of the restored wetlands [78] . We found that wetland restoration resulted in a significant reduction in the GWP (Table 1 ), mainly due to the substantial reduction in CO 2 emissions and the accompanying decrease of N 2 O emissions compared with the paired control ecosystems. Generally, wetland restoration could reduce GWP by 43-90% (Table S1 ). Among the wetland restoration measures, rewetting, moss layer transfer, and replanting & rewetting could significantly decrease GWP (Table S2 ). Returning croplands to wetlands is the most effective way to reduce GWP (Table S1 ). Our results were in accordance with the previous findings that wetland restoration remarkedly decreased GWP to a neutral range (3.3 to 6.7 t CO 2 -eq ha −1 yr −1 ) at the restored wetlands in comparison with the drained wetlands, mainly due to the increased CO 2 uptake by precluding oxidation of the residual in the restored wetlands [29] , [33] , [78] . Previous work found that the restoration of bogs through rewetting could yield exceptionally high CO 2 sink, which could effectively offset CH 4 emissions, thus resulting in a substantial reduction in the GWP [29] . Afforestation increased CH 4 and CO 2 uptake (Table 1 ), thus leading to a significant reduction in GWP with a mean of −10.3 t CO 2 -eq ha −1 yr −1 . Afforestation provided an effective strategy for GWP mitigation largely due to the increase in woody biomass C [82] . Grassland restoration resulted in a decrease in GWP across all the grassland types and restoration measures (Table 1 , Table S2 and S3 ), mainly by increasing the net CO 2 sink. Similarly, Rong et al. observed that grassland restoration brought about a greater increase in GPP than ER in a heavily grazed grassland, therefore decreasing NEE in the grassland [72] . Taking together, our study suggested that, forest, grassland, and wetland restoration could serve as an effective strategy for mitigating GHG emissions and reducing GWP. Implications for the IPCC reports, Guidelines for National Greenhouse Gas Inventories, and future research The present study provides a comprehensive understanding of the impacts of ecosystem restoration on GHG emissions at a global scale. Based on the compiled dataset, our results demonstrate that ecological restoration has vast potential to mitigate GHG at a global scale and provide insights and data for the IPCC reports and Guidelines for National Greenhouse Gas Inventories, particularly in relation to ecological restoration and land use change. In the context of “Agriculture, Forestry and Other Land Use (AFOLU)”, wetlands are recognized for their high level of uncertainty in the national greenhouse gas inventory reports submitted by States Parties to the United Nations Framework Convention on Climate Change (UNFCCC). Over the years, the IPCC has issued a series of methodological documents, such as “IPCC 2006 Guidelines for National Greenhouse Gas Inventories”, “2013 Supplement to the 2006 IPCC Guidelines for National Greenhouse Gas Inventories”, and “2019 Refinement to the 2006 IPCC Guidelines”. However, there is very little data regarding ecological restoration and its impacts on GHG emissions. The emission factors provided by the IPCC mainly focus on the dynamics of GHG in drained and rewetted organic soils [83] , [84] , [85] . Our study has expanded the available datasets for the restored wetlands and their paired control lands including different wetland types (bogs, mangroves, and floodplains wetland) and various land-use changes (i.e., conversion of cropland to wetland, conversion of grassland to wetland, conversion of forest to wetland, and returning aquaculture to wetland) (Figs. 3 , 4 ). In addition, our study provides an updated N 2 O emission factor for rewetted wetlands, estimated at 2.1 kg N ha ‒1 yr ‒1 (95% CI: 1.4 to 2.8) (Fig. 3d ), which is considerably higher than the assumed default value of 0 kg N ha ‒1 yr ‒1 for rewetted organic soils in the IPCC guidelines due to the limited data [79] . For the forests, the IPCC Guidelines only considered non-CO 2 gases from biomass burning and assumed that the conversion of croplands, grasslands and other lands to forest lands tended not to alter the sources and removals of non-CO 2 gases [85] . However, this assumption may not always hold true mainly due to the changes in soil properties resulting from land conversion (Fig. 6 and Supplementary Fig. S7 ) [12] , [21] . In our study, we conducted a detailed analysis for each land conversion type individually (i.e., conversion of croplands to forests and conversion of grasslands to forests) and developed a meta-data for non-CO 2 gases (i.e., CH 4 and N 2 O emissions) (Figs. 2 , 3 ), thereby providing valuable data for refining the non-CO 2 gases inventory methodology for the conversion of other lands into forests. 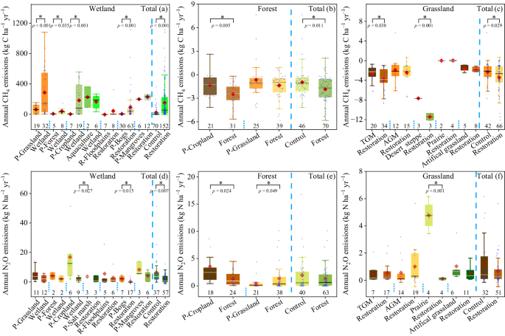Fig. 3: Box plots of CH4and N2O fluxes in the restored wetlands and their paired control ecosystems (a and d), the restored forests and their paired control ecosystems (b and e), the restored grasslands and their paired control ecosystems (c and f). Every two adjacent boxes represent the paired control-restored measurements. The paired control ecosystems are prefixed with ‘P’. TGM, temperate steppe & meadow; AGM, alpine steppe & meadow. Box boundaries represent the 75th and 25th percentiles, whisker caps represent the 95th and 5th percentiles, and circle points represent outliers. Diamond points and solid lines inside the boxes represent means and medians, respectively. Asterisks (*) denote significance atp< 0.05, as determined by using a two-sided, independent samplesttest. No adjustments were made for multiple comparisons. Numbers next to the x-axis indicate sample sizes (n). Exactp-values and Source data are provided as a Source Data file. Our results confirmed that afforestation and reforestation, as well as rewetting the drained wetlands, should become critical for future ecological restoration to mitigate GHG (Tables S1 and S2 , Fig. 5 ). In addition, previous work reported that the aquaculture systems are an important source of CH 4 [86] , and our results verified that returning aquaculture to wetlands was an effective measure to enhance C sinks (Table S1 ). Wetland restoration by converting drained forests, grasslands, and croplands into wetlands increased CO 2 sinks by decreasing ecosystem respiration, effectively transforming the ecosystems from CO 2 sources to sinks [29] . Bog restoration by rewetting can be an active restoration strategy to recover vegetation and convert the extracted bog from GHG sources to GHG sinks [26] (Table S2 ). For the grassland, restoring the degraded grassland either by grazing exclusion, reducing grazing intensity, or converting croplands to grassland is an effective strategy for mitigating GHG (Tables S2 and S3 ). These findings offer valuable insights for policymakers to select effective ecological restoration measures. Our study highlights the significance of restoration age in regulating GHG emissions in restored ecosystems, underscoring the importance of considering the time in assessing or modeling the effects of restoration or land-use change on GHG emissions (Fig. 5 and Supplementary Fig. S3 ). Although restoration measures can be implemented and completed quickly, the re-establishment of plant coverage and microbial communities is a gradual process [50] , [77] , [78] . The process of biomass accumulation changes over time [15] , [77] , and soil physical, biogeochemical, and hydrological properties change with restoration time [39] , [41] , [50] . Consequently, restoration age plays a significant role in regulating GHG budgets. Although biogeochemical processes in restored ecosystems have been studied in recent years [12] , [16] , [30] , [39] , there remains considerable uncertainty regarding the duration required for a restored ecosystem to transition into a net CO 2 sink. By compiling data from peer-reviewed literature, we identified the temporal patterns of NEE for forest and wetland restorations and determined the switchover time needed for the restored ecosystem to become a CO 2 sink. These temporal patterns of NEE highlighted the need for policymakers and planners to prioritize measures that facilitate the long-term recovery of the degraded systems in order to maximize climatic benefit and better achieve the goals of the UN Decade on Ecosystem Restoration (2021-2030). Moreover, the empirical equations and insights gained from our study regarding temporal patterns of NEE following restorations can provide important information for ecological modeling efforts. In addition, the soil CH 4 and N 2 O emissions are mainly governed by methanogens, methanotrophs, nitrifying and denitrifying microbes. However, studies about the effects of ecological restoration on these microbial communities are still insufficient [57] , [87] , which limits the explanation and prediction of the patterns of CH 4 and N 2 O emissions under ecological restoration. Therefore, future investigations should prioritize examining the microbial mechanisms underlying changes in soil CH 4 and N 2 O emissions during the ecological restoration process. 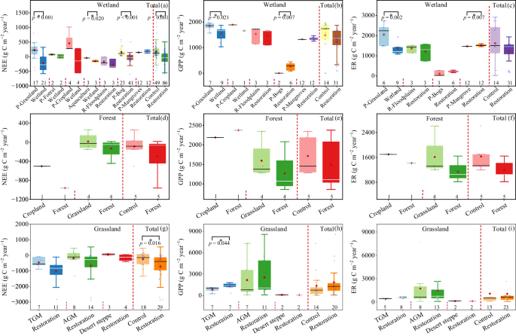Fig. 4: Box plots of annual CO2fluxes (NEE, GPP and ER) the restored wetlands and their paired control ecosystems (a–c), the restored forests and their paired control ecosystems (d–f), and the restored grasslands and their paired control ecosystems (g–i). Every two adjacent boxes represent the paired control-restored measurements. The paired control ecosystems are prefixed with ‘P’. Box boundaries represent the 75th and 25th percentiles, whisker caps represent the 95th and 5th percentiles, and circle points represent outliers. Diamond points and solid lines inside the boxes represent means and medians, respectively. Asterisks (*) denote significance atP< 0.05, as determined by using a two-sided, independent samplesttest. No adjustments were made for multiple comparisons. Numbers next to the x-axis indicate sample sizes (n). NEE net ecosystem CO2exchange, GPP, gross primary productivity, ER ecosystem respiration, TGM temperate steppe & meadow, AGM alpine steppe & meadow. Due to the small sample size for the paired restored-control measurements for the NEE, GPP, and ER in forests, the effects of forest restoration on CO2fluxes were not tested by the t-test. Exactp-values and Source data are provided as a Source Data file. Data source We compiled a global dataset on GHG emissions associated with ecological restoration from published literature (Fig. 1 ). We systematically searched the peer-reviewed literature from Google Scholar, Web of Science, and the China National Knowledge Infrastructure using the following keywords: TS = (restoration * OR rehabilitation * OR revegetation * OR recovery * OR reconstruction * OR reclamation * OR restored * OR restoring * OR recovering *) AND TS = (methane * OR CH 4 * or nitrous oxide * OR N 2 O * or carbon dioxide * OR CO 2 * or greenhouse gas *) AND TS = (wetland * or forest * or grassland *). The search results were filtered to include articles published between December 1999 and June 2023. Peer-reviewed studies were selected by the following criteria: (1) the selected experiments were conducted in the field from restored sites with paired control sites, or chronosequence sites; (2) each treatment was required to have at least three replicates; (3) the measurement covered an entire year or at least one growing season [88] ; (4) the selected studies reported at least one type of GHG. Finally, the dataset used in this study included a paired restored-control samples sub-dataset and a chronosequence sub-dataset, which were compiled from 253 peer-reviewed articles (Supplementary Fig. S8 ). The paired sub-dataset included 679 paired measured cases, and the chronosequence sub-dataset included 1289 data points with restoration age (i.e., years since restoration) (Supplementary Data 1 – 5 ). The dataset included: (1) GHG fluxes, including CH 4 , N 2 O, GPP, ER and NEE; (2) environmental factors, including longitude, latitude, mean annual air temperature (MAT), and mean annual precipitation (MAP); (3) restoration age, i.e., the years since restoration; (4) soil properties obtained from individual studies, including soil water table depth (WT), soil temperature (ST), and WFPS, Eh, BD, soil pH, SOC, TN, soil NH 4 + and soil NO 3 − . The fluxes of CH 4 , N 2 O and CO 2 were usually measured with the static chamber technique and eddy covariance method. The NEE is calculated as the differences of GPP and RE. If the GPP is lower than RE, then the NEE is positive, indicating net CO 2 sources to the atmosphere. In contrast, negative NEE indicates net CO 2 uptake from the atmosphere. The means, standard deviation (SD), and sample sizes for all variables in both restored and control ecosystems were extracted. If some studies (mainly eddy fluxes data) did not include SD values, SD was calculated as 1/10 of the mean [88] . Data in graphical figures and plots were extracted using Web Plot Digitizer (version 4.2). In this study, we used the definition of “ecological restoration” proposed by the Society for Ecological Restoration. Wetlands have been disturbed by human activities, including the draining of natural wetlands for croplands, grasslands and forests, the conversation of wetlands to aquaculture ponds, peatland extraction, floodplain drainage, mangroves deforestation, etc [3] , [76] . Wetland restoration is defined as the process of rebuilding the pre-disturbance ecosystem, including the biogeochemical and hydrological processes typical of water-saturated soils, as well as the recovery of vegetation to the former natural ecosystem [29] . According to the collected data in this study, the main types of wetland restoration included the following categories: (1) conversion of drained grasslands to wetlands, (2) conversion of drained croplands to wetlands, (3) conversion of drained forests to wetlands, (4) returning the aquaculture ponds to wetlands, (5) floodplain restoration by rewetting, (6) bog restoration by rewetting and moss layer transfer technique, and (7) mangroves restoration by planting. Based on the collected forest data that meet the selection criteria, forest restoration in this study included the conversion of grasslands to forests and the conversion of croplands to forests [43] . In addition, forest restoration from the disturbances (i.e., clear-cutting, fire and windstorm) was included in the chronosequence sub-dataset (Fig. 5 ). Grassland degradation was mainly due to overgrazing, land abandonment, or land conversion to croplands [89] . Thus, restoration measures included recovering degraded grassland via grazing exclusion, reducing grazing intensity, artificial assisted restoration, and conversion of croplands to grasslands. The types of grasslands were classified as prairies, temperate steppe & meadow (TGM), alpine steppe & meadow (AGM), and desert steppe (DS) [90] . Data analysis We used meta-analysis to examine the response of GHG and environmental factors to ecological restoration. Wetlands, forest and grassland ecosystems can both release CH 4 or CO 2 into the atmosphere (positive values) and uptake CH 4 or CO 2 into the atmosphere (negative values). Thus, the natural logarithm-transformed response ratio ( RR ) is not suitable for meta-analysis in our study. Here, Hedges’ d was used to evaluate the weighted response ratios ( RRd ) as it ranges from −∞ to +∞ [43] , [44] . The Hedges’ d was calculated as follows (Eq. 1 , Eq. 2 ): 
    RRd=(1-3/4(N_t+N_-2)-1)×X_t-X_c/S
 (1) 
    S=√((_-1)_^2+(_-1)_^2/_+_-2)
 (2) The variance ( vd ) was estimated with the following equation (Eq. 3 ): 
    vd=_+_/__+d^2/2(N_t+N_c )
 (3) where X t and Xc are the means of the concerned variable in the restored and paired control groups, respectively. S is the pooled standard deviation. N t and N c refer to the sample size of variables of the restored and paired control groups, and S t and S c are the corresponding standard deviation. MetaWin 3 software was used to calculate the overall effect size with a categorical random effects model [43] . Confidence intervals (95%; CIs) were calculated by bootstrapping (9999 iterations). The responses of variables to ecological restoration can be considered significant if the 95% confidence interval of the weighted effect size does not overlap zero (α = 0.05). If the 95% CI overlapped with zero, it assumed that there was no significant difference between the restored and paired control ecosystems. The effects of ecological restoration on the soil properties also were calculated using the above equations. To estimate the greenhouse effect of GHG emissions in ecosystems, GWP (t CO 2 -eq ha −1 year −1 ) from CH 4 , N 2 O and CO 2 fluxes (CH 4 and CO 2 : g C m −2 year −1 ; N 2 O: g N m −2 year −1 ) was calculated as follows (Eq. 4 ) [1] , [4] , [29] : 
    GWP=(27.2×16/12×CH_4+273×44/28×N_2O+44/12×NEE)× 100
 (4) where the fractions 16/12, 44/28 and 44/12 were used to transform the mass of C for CH 4 and CO 2 and nitrogen for the N 2 O to CO 2 equivalent, respectively [44] . 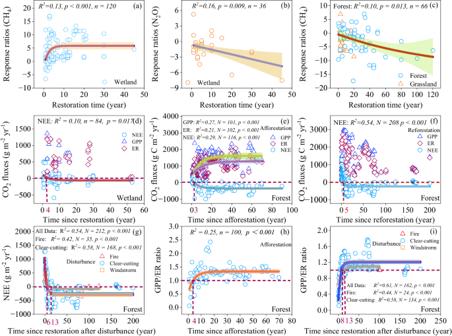Fig. 5: Relationships of the response ratios (RRd) of CH4and N2O fluxes, and the annual CO2fluxes with restoration age. a,brelationships between the response ratios of wetland CH4(a) and N2O (b) fluxes and restoration age.cRelationship between the response ratios of forest and grassland CH4fluxes and restoration age.d–frelationships between the CO2fluxes in wetland (d) and forest (eandf) and restoration age.grelationships between the fluxes of NEE and restoration age.h,irelationships between GPP/ER and afforestation time (h), and restoration age after forest disturbance (i). Linear and nonlinear regression were used and the error bands surrounding the regression lines represent the 95% confidence interval of the correlation. The n is the number of observations. Exactp-values and Source data are provided as a Source Data file. The 27.2 and 273 are the GWP values for CH 4 and N 2 O, respectively, to CO 2 over a 100-year time horizon [1] . One-way analysis of variance (ANOVA) was used to test the differences in GHG fluxes (CH 4 , N 2 O, GPP, NEE and ER) and soil variables between the restored and paired control ecosystems using IBM SPSS Statistical Tool (Version 23.0; SPSS Inc.). 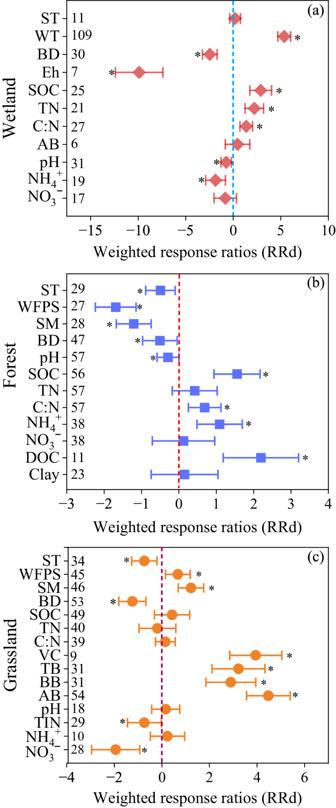Fig. 6: Effects of ecological restoration on soil properties in wetland (a), forest (b), and grassland (c) ecosystems. The overall effect size was calculated with a categorical random effects model. Values are meant ±95% CIs of the weighted response ratios (RRd) between the paired control ecosystems and restored ecosystems. If the 95% CI value does not overlap with zero, the response is considered significant. The asterisks indicate significant positive or negative effects. SOC soil organic carbon, TN total N, C: N carbon/nitrogen ratio, Eh soil redox potential, BD bulk density, SM soil moisture, WFPS water-filled pore space, ST soil temperature, WT water table depth, VC vegetation coverage, TB total biomass, AB aboveground biomass, BB belowground biomass; NH4+ammonium, NO3−nitrate. Source data are provided as a Source Data file. 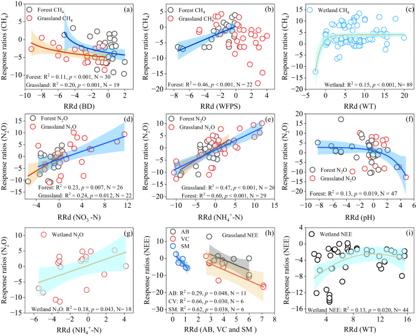Fig. 7: Relationships of the response ratios (RRd) of CH4(a–c), N2O (d–g), and NEE (h and i) with response ratios (RRd) of soil properties after wetlands, forest, and grassland ecosystems were restored. WT water table depth, BD bulk density, SM soil moisture, WFPS water-filled pore space, AB aboveground biomass, VC vegetation coverage. Linear and nonlinear regression were used and the error bands surrounding the regression lines represent the 95% confidence interval of the correlation. The n is the number of paired observations. Exactp-values and Source data are provided as a Source Data file. To explore the relationships between GHG fluxes and environmental factors, the mixed meta-regression was adopted after the calculation of the random effect model. In all statistical tests, the level of significance was set at P < 0.05. Reporting summary Further information on research design is available in the Nature Portfolio Reporting Summary linked to this article.